Alzheimer’s disease mutations in APP but not γ-secretase modulators affect epsilon-cleavage-dependent AICD production Pathological amino-acid substitutions in the amyloid precursor protein (APP) and chemical γ-secretase modulators affect the processing of APP by the γ-secretase complex and the production of the amyloid-beta peptide Aβ42, the accumulation of which is considered causative of Alzheimer’s disease. Here we demonstrate that mutations in the transmembrane domain of APP causing aggressive early-onset familial Alzheimer’s disease affect both γ- and ε-cleavage sites, by raising the Aβ42/40 ratio and inhibiting the production of AICD50–99, one of the two physiological APP intracellular domains (ICDs). This is in sharp contrast to γ-secretase modulators, which shift Aβ42 production towards the shorter Aβ38, but unequivocally spare the ε-site and APP- and Notch-ICDs production. Molecular simulations suggest that familial Alzheimer’s disease mutations modulate the flexibility of the APP transmembrane domain and the presentation of its γ-site, modifying at the same time, the solvation of the ε-site. The main pathological hallmark of Alzheimer’s disease (AD) is the formation of toxic amyloid fibres that progressively accumulate into plaques, which leads to degeneration of the neighbouring neuronal cells [1] . Further biochemical studies identified the main protein component of plaques to be a short fragment of amyloid precursor protein (APP), the 42-amino acid long peptide Aβ42 (ref. 2 ). Moreover, dominantly inherited mutations causing familial Alzheimer’s disease (FAD) are found in APP as well as in the PSEN1 and PSEN2 (refs 3 , 4 ) genes encoding for the catalytic subunit of the γ-secretase complex, an intramembrane-cleaving protease that cleaves APP in the plasma membrane and generates the Aβ peptides [5] . Together, these findings clearly demonstrated the implication of APP, γ-secretase and Aβ in both the sporadic and genetic forms of AD. They further highlighted the γ-secretase-dependent APP processing as an attractive target for drug development. In addition to APP, γ-secretase cleaves various other substrates regulating biological functions including development and stem cell differentiation. This unusual proteolytic complex indeed has an important role in cell signalling pathways by processing different type-I transmembrane cell receptors including the Notch receptors, the Insulin receptor and the Growth hormone receptor [6] . In the brain, it maintains synaptic contacts by regulating cleavage of neuronal adhesion molecules like Cadherins and Neurexins [7] , [8] . With the continuously growing number of substrates the need for understanding the exact molecular mechanism of this particular proteolytic processing arises. γ-Secretase is composed of four subunits, presenilin (PS), Aph-1, Pen-2 and Nicastrin (NCT). The complex contains a total of 19 α-helices embedded in the membrane bilayer, which allows the overall structure to adopt different conformations upon binding with the substrate or different chemical compounds [9] , [10] . Moreover, the catalytic aspartate residues (Asp257/385) in hPS1 are buried into the lipid bilayer and surrounded by hydrophobic helices and the electron microscopy density maps suggested the existence of two pores in the globular structure of γ-secretase, which can explain the entrance of water molecules necessary for the hydrolysis of the peptide bond [11] . Yet, a rigorous biochemical characterization of γ-secretase complexes with FAD mutations revealed that they all represent a loss of enzymatic function, but they ultimately lead to altered Aβ production and elevated Aβ42/40 ratio [12] , [13] . Interestingly, FAD mutations in APP can show substrate cleavage patterns that differ from those of the mutations in γ-secretase. In the processing of APP, its large extracellular domain is first removed by β-secretase in the vicinity of the plasma membrane ( Fig. 1 ). Gain-of-function mutations in this β-site cause elevated levels of total Aβ [14] . γ-Secretase processes the remaining 99-amino-acid APP-C-terminal fragment (APP-C99) at ε-sites close to the inner layer of the membrane, and releases 49- and 50-amino-acid long APP intracellular domains (AICD50–99 and AICD49–99; Fig. 1 ). After this step, γ-secretase sequentially continues to trim the residual transmembrane stub, finally producing Aβ42, Aβ40 and Aβ38 peptides [15] ( Fig. 1 ). Mutations surrounding the ε-sites either increase the production of Aβ42, which is more neurotoxic compared to the shorter and less fibrillogenic Aβ40 or lead to elevated total amounts of the Aβ product without affecting Aβ ratios [13] , [16] . Amino-acid substitutions in the γ-site lead to high Aβ42/40 ratios and are characterized by the most prominent and earliest phenotypes of FAD [17] . 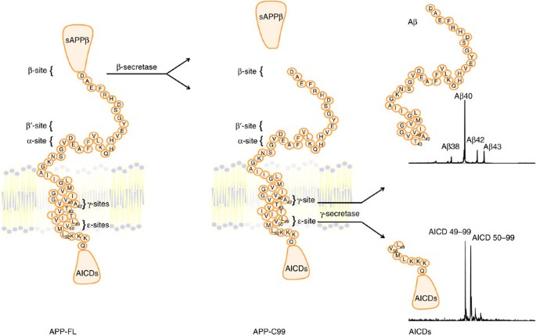Figure 1: Sequential proteolytic processing of APP by β- and γ-secretases. Full-length APP is initially cleaved by β-secretase, liberating a soluble APPβ (sAPPβ) into the extracellular space. The remaining 99-amino-acid long transmembrane APP-C99 is further processed by γ-secretase at ε-sites, close to the inner layer of the membrane, releasing two APP intracellular signalling domains (AICDs) differing by one amino acid in length, AICD49–99 and AICD50–99. These products are in nearly equimolar ratio as depicted in the representative mass spectrometry AICD profile. Next, γ-secretase continues to trim the residual membrane-embedded N-terminal fragment at γ-sites, finally generating Aβ peptides secreted into the extracellular space. In contrast to equimolar AICD production, mass spectrometric analysis of secreted Aβ shows that Aβ40 is in large excess when compared to the more amyloidogenic Aβ42 directly involved in the pathogenesis of AD through the formation of Aβ plaques. Figure 1: Sequential proteolytic processing of APP by β- and γ-secretases. Full-length APP is initially cleaved by β-secretase, liberating a soluble APPβ (sAPPβ) into the extracellular space. The remaining 99-amino-acid long transmembrane APP-C99 is further processed by γ-secretase at ε-sites, close to the inner layer of the membrane, releasing two APP intracellular signalling domains (AICDs) differing by one amino acid in length, AICD49–99 and AICD50–99. These products are in nearly equimolar ratio as depicted in the representative mass spectrometry AICD profile. Next, γ-secretase continues to trim the residual membrane-embedded N-terminal fragment at γ-sites, finally generating Aβ peptides secreted into the extracellular space. In contrast to equimolar AICD production, mass spectrometric analysis of secreted Aβ shows that Aβ40 is in large excess when compared to the more amyloidogenic Aβ42 directly involved in the pathogenesis of AD through the formation of Aβ plaques. Full size image Inhibiting the γ-secretase activity to reduce Aβ production is an attractive therapeutic strategy to treat AD. However, γ-secretase inhibitors (GSIs) tested in clinical trials not only failed to meet their initial clinical endpoints, but also manifested severe off-target effects due to impaired Notch signalling, leading to gastrointestinal bleeding and increased risk of skin cancer [18] . Consequently, a concept of selective modulation of the γ-secretase activity has emerged. A subset of non-steroidal anti-inflammatory drugs (NSAIDs) were the first Notch-sparing small molecules shown to selectively lower Aβ42 and subsequently raise Aβ38 both in vitro and in vivo [19] , [20] . These γ-secretase modulators (GSMs) were initially shown to bind to APP, although some more recent studies demonstrated that they also can target γ-secretase [21] , [22] . Although the precise molecular mechanism of action remains poorly understood, a number of these molecules have advanced to clinical trials [23] . In this report, we demonstrate that second generation GSMs, including the clinically tested E2012, effectively lower the production of toxic Aβ42 without affecting the ε-cleavage sites of both APP and Notch substrates. In contrast, we show that the T714I, V715A, V717F and L723P FAD-APP mutations in the transmembrane (TM) region block the production of AICD50–99, the 49-amino-acid long AICD, without affecting the total amount of AICD. Moreover, mutations T714I and V715A elevate the Aβ42/40 and Aβ38/40 ratios, in contrast to I716V, V717F and L723P for which these profiles were comparable to those obtained with wild-type APP. GSMs affect all mutants at their γ-cleavage site, with the strongest effect on the Aβ38/40 and Aβ42/40 ratios in T714I and V715A, suggesting that these amino-acid substitutions are important for the generation of Aβ42 and Aβ38. In addition, we find that GSMs do not reverse the loss of AICD50–99 production caused by FAD mutations. We rationalize these findings using molecular dynamic simulations of the APP TM segment embedded in the lipid bilayer, and propose that FAD-APP mutants and possibly GSMs affect the γ-cleavage site by changing the flexibility, tilt angle and position of the substrate in the membrane. GSMs fail to recover ε-cleavage, most likely because they affect the substrate–enzyme interface at a position that is distant from the ε-site and closer to the outer layer of the membrane. Finally, FAD mutants have altered solvation at the ε-cleavage site, which can explain the different product lines generated after the first step of the processing of APP. GSMs affect the γ- but not the ε-cleavage of APP and Notch We first investigated the effect of GSM-1 and E2012, two representative molecules of the two main classes of second generation GSMs: NSAID-based phenylpiperidine-type compounds and non-NSAID bridged aromatics, respectively ( Fig. 2a ). Although these compounds have different structures, they both modulate γ-secretase activity at low nanomolar concentrations in cells [24] . In enzymatic in vitro assays using highly purified γ-secretase and recombinant APP-C100-Flag substrate, we first show that concentrations several fold higher than the cellular IC 50 values of GSM-1 and E2012 do not affect the overall amounts of Aβ and AICD, when compared to control levels ( Fig. 2b , upper panels and Supplementary Fig. S1 ). We next investigated in detail the effect of these molecules on all reaction products. For both compounds tested at 10 μM, immunoprecipitation with 4G8 anti-Aβ antibody, combined with MALDI-TOF spectrometry (IP/MS) revealed a robust increase of Aβ38/40 ratio, associated with a decrease in Aβ42/40 ratio ( Fig. 2b , middle panels). At this concentration, GSM-1 showed a stronger effect than E2012 on Aβ42/40 and Aβ38/40 ratios, while both compounds lowered Aβ43/40 ratio. IP/MS analyses of the C-terminal cleavage products revealed an unchanged equimolar production of the two AICDs ( Fig. 2b , lower panels). Together, these results clearly demonstrate that GSMs affect the APP γ-cleavage sites, whereas they completely spare the ε-sites. Because of the clinical relevance of GSMs and the Notch signalling pathway, we further investigated whether GSMs could interfere with the Notch intracellular domain (NICD) production. As shown in Fig. 2c , GSMs did not influence total NICD production and did not affect the NICD cleavage profiles. Our in vitro findings were further confirmed in cell-based assays. First, intracellular accumulation of endogenous γ-secretase substrates APP-C83 and APP-C99, which is a common characteristic among known γ-secretase substrates in response to γ-secretase inhibition, was assessed in HEK293T cells stably overexpressing APP with the FAD Swedish mutation KM670/671NL. In contrast to the control GSI, 1 and 10 μM E2012 or GSM-1 did not affect the levels of APP-CTFs ( Supplementary Fig. S2a ). Next, treatments with E2012 and GSM-1 up to 1 μM in a cell-based luciferase assay, in which AICD generation correlates with increased luciferase expression and induced luminescence emission, did not result in a significant inhibition of AICD release ( Supplementary Fig. S2b ). Additionally, the GSMs were tested in human lymphocytic leukaemia SUP-T1 cells constitutively producing NICD. In contrast to the GSI XIX that completely abolished NICD production, E2012 and GSM-1 did not affect NICD production at concentrations up to 10 μM ( Supplementary Fig. S3a ). These findings were confirmed in a cellular Notch-based assay in which a luciferase reporter system is directly placed under the control of NICD ( Supplementary Fig. S3b ), as well as in RPMI8402 (ref. 25 ) cells expressing a mutated Notch-1 receptor, which makes the receptor susceptible to constitutive cleavage by γ-secretase in a ligand-independent manner ( Supplementary Fig. S3c ). In the latter two assays, E2012 and GSM-1 concentrations up to 1 μM did not affect NICD production. At 10 μM, E2012, but not GSM-1, significantly reduced NICD production in DL4-Hela/N1-Hela co-cultures by 55% (*** P <0.001, Supplementary Fig. S3b ). Taken together, we conclude that E2012 and GSM-1 do not alter the Notch and APP ε-site cleavage at concentrations as high as 10-fold cellular IC 50 . At higher concentrations (~100-fold cellular IC 50 ), only the non-NSAID-based compound E2012 can inhibit to some extent intracellular signalling of Notch and APP in cell-based assays. 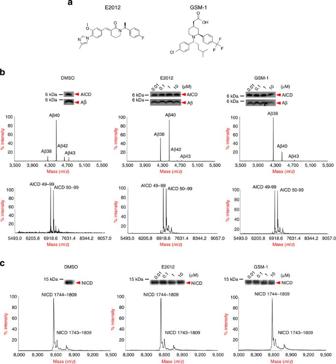Figure 2: GSMs alter γ-site processing but do not modulate ε-site on APP-C99-Flag and NotchΔE-Flagin vitroby highly purified γ-secretase. (a) Chemical structure of clinically tested small molecules NSAID-based phenylpiperidine-type GSM-1 and bridged aromatics E2012. (b) GSMs do not inhibit the overall cell-free processing of APP-C99-Flag as shown by WB analysis of Aβ and AICD at concentrations ranging from low nanomolar to low micromolar. Following immunoprecipitation, analysis by MALDI-TOF demonstrated the efficacy of GSMs on the γ-site, where they shifted the production towards shorter Aβ38 and lowered Aβ42. Even at concentrations as high as 10 μM, GSMs do not alter the ε-site as evidenced by the IP/MS on the AICD products, AICD49–99 and AICD50–99. (c) GSMs show no inhibition on Notch intracellular signalling products.In vitroNICD formation from NotchΔE-Flag as detected by WB is unaltered. The ratio of the two NICD products, NICD1744-1809 and NICD1743-1809, detected after IP/MS, also remained without change in the presence of 10 μM of both compounds. Figure 2: GSMs alter γ-site processing but do not modulate ε-site on APP-C99-Flag and NotchΔE-Flag in vitro by highly purified γ-secretase. ( a ) Chemical structure of clinically tested small molecules NSAID-based phenylpiperidine-type GSM-1 and bridged aromatics E2012. ( b ) GSMs do not inhibit the overall cell-free processing of APP-C99-Flag as shown by WB analysis of Aβ and AICD at concentrations ranging from low nanomolar to low micromolar. Following immunoprecipitation, analysis by MALDI-TOF demonstrated the efficacy of GSMs on the γ-site, where they shifted the production towards shorter Aβ38 and lowered Aβ42. Even at concentrations as high as 10 μM, GSMs do not alter the ε-site as evidenced by the IP/MS on the AICD products, AICD49–99 and AICD50–99. ( c ) GSMs show no inhibition on Notch intracellular signalling products. In vitro NICD formation from NotchΔE-Flag as detected by WB is unaltered. The ratio of the two NICD products, NICD1744-1809 and NICD1743-1809, detected after IP/MS, also remained without change in the presence of 10 μM of both compounds. Full size image APP mutations differentially alter γ- and ε-sites APP mutations causing FAD can be grouped based on their localization at three different regions: at the β-secretase cleavage site, in close vicinity of the α-secretase cleavage site in the Aβ region or in the transmembrane domain (TMD) of APP, between the γ- and the ε-sites ( Fig. 3a , left). These mutations differ not only by the onset of the disease ( Fig. 3a , right), but also by the molecular fingerprint of the produced Aβ peptides. Indeed, the vast majority of mutations in the α-and β-sites lead to the overproduction of total Aβ (mutations in the Aβ region can also render the Aβ42 peptide more fibrinogenic and prone to aggregation), while mutations in the transmembrane region seem to be linked to an elevated Aβ42/40 ratio [13] , [26] . As no information exists about how these mutations affect both the γ- and ε-cleavage sites in APP, and because AICD has been suspected to have a role in the pathogenesis of AD, we analysed Aβ and AICD products generated from purified His6-tagged APP-C99 substrates carrying the FAD mutations listed in Fig. 3a . As shown in Supplementary Figs S4 and S5 , we first verified that His6- and Flag-tagged substrates respond to GSM treatments in an identical manner, confirming that different tags (His6 or Flag) do not affect either the profiles of γ- and ε-site products ( Supplementary Fig. S4 ), or the overall production of Aβ or AICD ( Supplementary Fig. S5 ). Next, IP/MS analyses of the Aβ and AICD profiles revealed that amino-acid substitutions clustered near the α-secretase (A692G, E693G and D694N) apparently do not alter the Aβ or AICD profiles, when compared to the control WT APP-C99 ( Fig. 3b and Table 1 ). In striking contrast, T714I and V715A mutations close to the transmembrane γ-cleavage site lead to drastically increased Aβ42/40 and Aβ38/40 ratios and to a total inhibition of the production of the shortest AICD50–99 ( Fig. 3b,c and Table 1 ). Interestingly, mutations closer to the ε-cleavage sites (I716V, V717F and L723P) are characterized by an intermediate phenotype as they do not alter Aβ profiles, but clearly lower the production of AICD50–99 (below detection levels for V717F and L723P; Fig. 3b,c and Table 1 ). Taken together, our data demonstrate that FAD-causing mutations in the transmembrane region of APP, but not close to the α-secretase site, affect both γ- and/or ε-sites (summarized in Table 1 ). 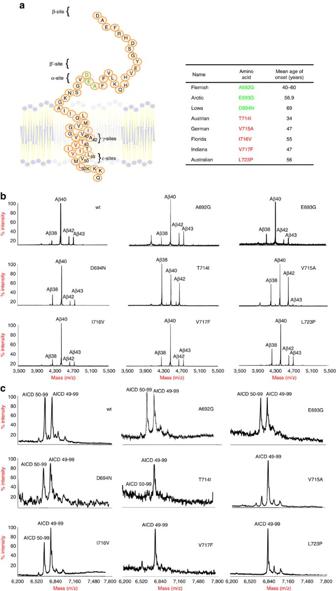Figure 3: Pathological mutations in APP cause altered processing at both ε- and γ-sites. (a) FAD-APP mutations differ by the onset, but are all clustered close to the α-secretase and γ-secretase cleavage sites, as represented schematically in the left panel (colour coding: α-secretase site mutations in green; γ-secretase site mutations in red). Different mean onsets are summarized in the right table. The earliest onset is reported for Austrian and German families at the age of 34 and 47 years, respectively. (b) IP/MS profiles of Aβ generated from purified His-tagged FAD-APP-C99 substrates show that mutations A692G, E693G, D694N, I716V, V717F and L723P have similar and WT-like Aβ38/40 and Aβ42/40 ratios. In contrast, T714I and V715A mutations in the transmembrane region led to a drastic increase in both Aβ38/40 and Aβ42/40 ratios. (c) AICD profiles from the same reactions as analysed by IP/MS. FAD-APP-C99 mutations close to the α-secretase site produce AICD49–99 and AICD50–99 in nearly equimolar ratios. Amino-acid substitutions in close vicinity of the γ-sites in the TMD strongly affect the yield of shorter AICD50–99. Figure 3: Pathological mutations in APP cause altered processing at both ε- and γ-sites. ( a ) FAD-APP mutations differ by the onset, but are all clustered close to the α-secretase and γ-secretase cleavage sites, as represented schematically in the left panel (colour coding: α-secretase site mutations in green; γ-secretase site mutations in red). Different mean onsets are summarized in the right table. The earliest onset is reported for Austrian and German families at the age of 34 and 47 years, respectively. ( b ) IP/MS profiles of Aβ generated from purified His-tagged FAD-APP-C99 substrates show that mutations A692G, E693G, D694N, I716V, V717F and L723P have similar and WT-like Aβ38/40 and Aβ42/40 ratios. In contrast, T714I and V715A mutations in the transmembrane region led to a drastic increase in both Aβ38/40 and Aβ42/40 ratios. ( c ) AICD profiles from the same reactions as analysed by IP/MS. FAD-APP-C99 mutations close to the α-secretase site produce AICD49–99 and AICD50–99 in nearly equimolar ratios. Amino-acid substitutions in close vicinity of the γ-sites in the TMD strongly affect the yield of shorter AICD50–99. Full size image Table 1 Summary of the apparent ratios from the different γ - and ε -site products. Full size table GSMs affect the γ- but not the ε-cleavage of APP To better understand the molecular mechanism by which GSMs shift Aβ production, as well as to verify whether GSMs can still lower Aβ42 and have potential therapeutic benefits in patients with FAD, we decided to test GSM-1 on APP-C99 with FAD mutations. GSM-1 was chosen because it was more potent in our in vitro γ-secretase assay, and also because this compound did not affect ε-cleavage in all cell-based experiments. First, 10 μM GSM-1 did not affect the levels of total cleavage products (compare AICD and Aβ levels in Supplementary Figs S4a and S5b ), providing further evidence that GSMs do not modify the overall yield of γ-secretase processing. Next, we found that GSM-1 conserved its Aβ42-lowering and Aβ38-raising properties on all tested mutant substrates ( Fig. 4a ). However, GSM-1 did not influence the ε-cleavage and none of the mutants tested recovered the wild-type phenotype of nearly equimolar production of AICD49–99 and AICD50–99 (compare AICD profiles in Figs 4b and 3c , and see estimations of AICD 49–99/AICD50–99 ratios in Table 2 ). Our findings provide new evidence that GSMs lower Aβ42/40 ratio production by interfering with the γ-site in APP substrates with FAD mutations, strongly suggesting that none of the substituted amino-acid residues are crucial for the GSM-dependent modulation of APP processing by γ-secretase. They further demonstrate that GSMs do not affect the ε-cleavage site and thus fail to reverse the effects on AICD production of FAD-causing mutations in the transmembrane domain of APP (summarized in Table 2 ). 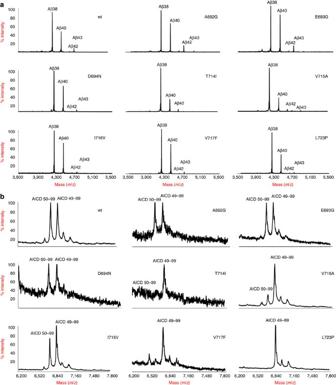Figure 4: GSMs potently shift the production at γ- and not at ε-sites in APP with FAD mutations. (a) IP/MS profiles of Aβ species produced from purified His-tagged APP-C99 substrates with FAD mutations, demonstrate the efficacy of GSMs towards the γ-site processing. For all FAD-APP mutants tested, Aβ38/40 and Aβ42/40 ratios are strongly affected by 10 μM of GSM-1. Mutations T714I and V715A had the most elevated Aβ38/40, implying that amino acids between APP γ- and ε-sites are not essential for the GSM mechanism of action. (b) IP/MS profiles of the ε-site products from the same reactions provide supplementary evidence that GSMs do not influence the ε-sites in APP. Even high concentrations of GSM-1 fail to restore the loss of shorter AICD50–99 in mutants T714I, V715A, V717F and L723P. Figure 4: GSMs potently shift the production at γ- and not at ε-sites in APP with FAD mutations. ( a ) IP/MS profiles of Aβ species produced from purified His-tagged APP-C99 substrates with FAD mutations, demonstrate the efficacy of GSMs towards the γ-site processing. For all FAD-APP mutants tested, Aβ38/40 and Aβ42/40 ratios are strongly affected by 10 μM of GSM-1. Mutations T714I and V715A had the most elevated Aβ38/40, implying that amino acids between APP γ- and ε-sites are not essential for the GSM mechanism of action. ( b ) IP/MS profiles of the ε-site products from the same reactions provide supplementary evidence that GSMs do not influence the ε-sites in APP. Even high concentrations of GSM-1 fail to restore the loss of shorter AICD50–99 in mutants T714I, V715A, V717F and L723P. Full size image Table 2 Summary of the apparent ratios from the different γ- and ε-site products. Full size table Structural changes in the TM domain of APP To support our results mechanistically, we used molecular dynamic (MD) simulations to gain further insights into the structural and dynamic properties of the TMD of wild-type APP and three FAD mutants (T714I, V715A and V717F) in the membrane environment. These mutations were chosen because they affect either both γ- and ε-cleavage sites (T714I and V715A), or exclusively the ε-site (V717F). As γ-secretase activity assays performed with purified enzyme and APP-C99 substrate reconstituted in PC+PE (phosphatidyl choline and phophatidylethanolamine) or PC alone revealed almost identical IP/MS profiles of Aβ and AICDs ( Supplementary Fig. S6 ), the TM region of the APP-C99 NMR structure (PDB code 2LP1 (ref. 27 )) was used and inserted into a palmitoyl oleoyl phosphatidylcholine (POPC) lipid bilayer ( Fig. 5a ). Thus, MD simulations were carried out under physiological-like conditions (that is, pH~7, 1 atm, 300 K), mimicking as closely as possible the conditions of the γ-secretase enzymatic assay used in our study. For all systems, the secondary structure of the APP fluctuated only marginally. Consistent with the NMR observations, the N terminus amphiphilic helix (Q686–N698) lies on the membrane surface, whereas a lysine belt (K687, K699 and K724–726) anchors the TMD and N terminus helices, respectively, in and onto the membrane ( Fig. 5a ). During simulation, the helices tilted with respect to the membrane surface. We found that the V717F mutation affected the orientation of the TMD the most, tilting it by 45±5°, whereas the wild type and T714I and V715A mutants remained more vertical (36±5°, 38±3° and 36±3°, respectively) ( Fig. 5a and Supplementary Fig. S7a ). These mutations further shifted the TMD perpendicularly to the membrane surface. When measuring the position of the Aβ42 cleavage site (that is, I712–A713 peptide bond), the T714I and V715A mutants shifted closer (2.9±1.2 Å and 2.3±0.9 Å, respectively) to the cytoplasmic interface compared to the WT, whereas V717F moved closer (−0.2±1.3 Å) to the extracellular membrane layer ( Fig. 5b ). The combined effect of shifting and tilting perturbations of the APP TMD is due to FAD mutations. This probably affects the presentation of the γ-cleavage site at position 42 to the enzyme and correlates quantitatively with the changes in the Aβ42/Aβ40 ratio. Moreover, the flexibility of the transmembrane domain, which was estimated based on the local bending of the helix [28] , was much higher for the T714I and V715A mutants, specifically at the G 700 XXXG 704 XXXG 708 region ( Fig. 5c ). Molecular docking and simulations of the GSM-1 compound suggest the same region to be the conserved drug-binding pocket for the wild-type and mutant APPs ( Supplementary Fig. S7b ). In the drug-binding pocket, L701, G704 and G708 had the most direct interactions with GSM-1. Thus, the effect of GSM-1 on T714I and V715A FAD mutants might cause a reduction of their flexibility close to the γ-site. For all three mutants, the hydration of the ε-site at residue L720 significantly decreased compared to the WT ( Fig. 5d ). In particular, for APP-WT, one water molecule is on an average within 3 Å of L720 backbone, the water coordination number drops to <0.5 Å for V715A, and to nearly zero for T714I and V717F. This effect is related to the different water permeation properties of the APP C terminus lysine belt combined with the perturbed helical orientation produced by the mutants. In summary, our data support a model in which structural changes, particularly the position of the γ-cleavage site relative to the membrane surface, can potentially modulate Aβ production. In this model the hydration of L720 can affect the ε-cleavage site and the production of the two amyloid precursor protein intracellular domains potentially implicated in signalling pathways and in the pathogenesis of AD. 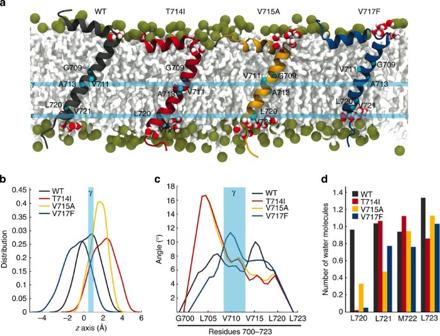Figure 5: Structural and dynamic models of the TM domain in WT and FAD-causing APP mutants. (a) The NMR structure of WT APP (PDB code:2LP1(ref.28)) and three FAD-causing mutants, namely T714I, V715A and V717F, were inserted in a POPC membrane bilayer and simulated with molecular dynamics. The γ-sites G709, V711 and A713 and ε-sites L720 and V721 positions are indicated by blue spheres. (b) The spatial distribution of Aβ42 cleavage site is reported for the four systems. The distribution is calculated along the axis orthogonal to the membrane bilayer surface and the reference putative position of the γ-site in wild-type conditions is highlighted with the blue area. (c) The local bending of the APP helix is computed for the TM domain (with a standard error of 2.8 degrees). (d) The coordination number of water molecules around the relevant residues at the ε-site is reported for the WT and mutants. Figure 5: Structural and dynamic models of the TM domain in WT and FAD-causing APP mutants. ( a ) The NMR structure of WT APP (PDB code: 2LP1 (ref. 28 )) and three FAD-causing mutants, namely T714I, V715A and V717F, were inserted in a POPC membrane bilayer and simulated with molecular dynamics. The γ-sites G709, V711 and A713 and ε-sites L720 and V721 positions are indicated by blue spheres. ( b ) The spatial distribution of Aβ42 cleavage site is reported for the four systems. The distribution is calculated along the axis orthogonal to the membrane bilayer surface and the reference putative position of the γ-site in wild-type conditions is highlighted with the blue area. ( c ) The local bending of the APP helix is computed for the TM domain (with a standard error of 2.8 degrees). ( d ) The coordination number of water molecules around the relevant residues at the ε-site is reported for the WT and mutants. Full size image Mutations in APP cause aggressive early-onset AD by triggering abnormal production, accumulation and aggregation of Aβ peptides. The most severe pathological phenotype is observed for mutations occurring in the transmembrane region and in close vicinity of the Aβ42 γ-cleavage site, leading to elevated Aβ42/40 and Aβ38/40 ratios ( Fig. 3 ). Small chemical γ-GSMs are known to lower Aβ42 and raise Aβ38, without affecting the overall production of the Aβ peptides. In this study, we used second generation GSMs with a strong therapeutic potential (GSM-1 and E2012), in combination with APP substrates with FAD-causing mutations, to better understand the molecular mechanisms of the γ-secretase-dependent, intramembrane and sequential cleavage of the substrate; to identify changes in APP cleavage profiles, potentially implicated in the pathogenesis of AD; and to further support the therapeutic potential of GSMs to safely treat sporadic as well as early-onset familial AD. We further demonstrate here that GSMs represent an attractive scaffold for structure–activity relationship design of potent disease-modifying drugs against AD. As they do not affect the processing of the Notch substrate ( Fig. 2 ), GSMs are expected to circumvent clinical side effects observed with GSIs and attributed to impaired Notch processing [18] . Moreover GSMs do not alter AICD production ( Fig. 2 ) and thus are not likely to influence the downstream cell signalling functions of APP, again underlying the huge therapeutic potential of these compounds in sporadic AD cases. Additionally, our results confirm altered γ-site processing in APP T714I and V715A mutations [13] , associated with an increase of Aβ42/40 and Aβ38/40 ratios and demonstrate that mutations located in close vicinity to the γ-site do impede the production of the shorter ε-site counterpart AICD50–99. Our novel findings shed light on the effect of GSMs on the generation of all Aβ and AICD species from APP-WT and APP-FAD. In our study, we have further investigated the effect of GSMs on the γ- and ε-site APP cleavage products. Our results show that none of the amino-acid residues of APP-WT causing FAD when mutated are critically implicated in the mechanism of action of GSMs in shifting the production from Aβ42 to Aβ38. Next, we demonstrate that GSMs are not involved in the first step of the sequential proteolytic model [15] because they do not modulate the ε-site products (AICD50–99 and AICD49–99) of the enzymatic reaction. Interestingly, mutations T714I and V715A display the strongest phenotype at both γ- and ε-sites, with highest Aβ42/40 and Aβ38/40 ratios ( Table 1 ). Moreover, these mutations lead to the production of only one detectable AICD, suggesting a putative role of AICD in AD pathogenesis. These results might be explained with the sequential cleavage model of APP-CTF, in which the generation of Aβ40 is dependent on the AICD50–99, while Aβ42/38 is linked to AICD49–99 (ref. 15 ). Based on this model, reduced AICD50–99 (as observed for some FAD mutants) is expected to be associated with less Aβ40 and more Aβ42/38, thus increasing the pathogenic ratio of Aβ42/40. The combination of higher Aβ42/40 ratio and the loss of AICD50–99 can explain the extreme aggressiveness of these APP mutations with regard to the onset of the disease. GSMs were still potent at the γ-site of mutated APP substrates ( Fig. 4 ), as expected from molecular docking and simulations suggesting the G 700 XXXG 704 XXXG 708 region as a possible GSM-binding pocket ( Supplementary Fig. S7b ). GSMs have also been shown to target PS1-NTF [9] , [22] , [29] , supporting the hypothesis that these compounds could bind at the interface between APP-C99 and the substrate-docking site of γ-secretase. Moreover, the region between γ- and ε-sites on APP-CTF has been proposed to be a binding domain for PS1-NTF [30] , and peptides mimicking this domain can selectively block Aβ production, sparing Notch processing [31] . Together, these findings clearly demonstrate that GSMs can be used for the treatment of patients with both sporadic and genetic forms of AD. Rationalizing these results with structural models based on molecular simulations of wild-type and mutant APP substrates, we propose that the observed effects on Aβ and AICD production can be triggered by combined changes in the flexibility, tilting angle and positioning of both γ- and ε-sites in the membrane, along with the hydration levels at the ε-sites. Such structural changes, by potentially modifying the presentation of the substrates to the enzymatic complex, might affect the γ-secretase cleavage specificity. Consistent with this model, the elevated Aβ38/40 ratio observed in mutants T714I and V715A can be explained by the vertical shift of the helix in the membrane bilayer, with the consequent presentation of position 38 instead of 40 to the γ-secretase cleavage site. The observed vertical shift in mutants (~2.5 Å) is in fact associated with a tilting of half of a helix turn (that is, displacement of two amino acids). Interestingly, Aβ38 and Aβ42 have been proposed to originate from the same sequential processing pathway, starting at the ε-position 48, and directly linked to AICD49–99 production [15] . Consistent with this sequential model, we propose that the conformational changes in the T714I and V715A substrates, associated with reduced AICD50–99 levels, explain the preferential Aβ38 and Aβ42 production observed with these mutants. Interestingly, and apparently in contrast to the sequential cleavage model, the V717F and L723P mutants, although characterized by reduced AICD50–99 levels, do not show modifications in their Aβ profiles. This observation may reflect the existence of two or more different pathological molecular explanations, classifying FAD forms in different categories. The nearly complete loss of AICD50–99 production in mutants T714I, V715A, V71F and L723P, can plausibly be attributed, according to our model, to higher solvation states around positions 49 and 50, with the latter becoming more exposed to water molecules. One can speculate that the increased water accessibility to the leucine 49 may favour the cleavage at this position, or inhibit the cleavage at valine 50 by preventing the interaction at position 50 of APP-C99 with the hydrophobic transmembrane domain 1 of the γ-secretase catalytic component PS1. Possibly affecting the positioning of both APP γ- and ε-sites in the membrane, cholesterol and the dimerization of APP have recently been proposed to modulate the processing of APP-TMD [32] , [33] . Although preliminary, our results ( Supplementary Fig. S8 ) suggest that when APP does not interact physically with cholesterol molecules in a membrane made of POPC+15% cholesterol, the dynamic properties of its TMD, including the position of the Aβ42 cleavage site, are the same as those of APP inserted into a pure POPC membrane. Further investigation is required to challenge this hypothesis, and examine whether both cholesterol levels and APP dimerization parameters can affect the dynamic properties of wt or FAD-APP TMDs. Together, our data reported here provide new insights into the therapeutic potential of chemical γ-secretase modulators. They are further expected to improve our current understanding of the pathological mechanism of FAD. γ-Secretase inhibitors and modulators γ-Secretase inhibitors Compound E and GSI XIX were purchased from Merck Millipore (Darmstadt, Germany). The heteroaryl-type GSM E2012 (US2006/0004013) was obtained from Haoyuan Chemexpress Co and the NSAID-type GSM-1 was synthesized at Syngene according to methods described in WO2006/043064. Molecular biology The pET21b vector encoding the cDNAs of human APP-C100-His was used as a template for the generation by PCR amplification of all His6-tagged FAD-APP-C100 mutants described in this study. The constructs were expressed in BL21(DE3) cells induced with 1 mM isopropyl-β-D-thiogalactopyranoside (IPTG) for 4 h at optical density 600 nm=0.8. For the purification of APP-C99 mutants, harvested bacteria were lysed with 10 mM Tris (pH 7.0), 150 mM NaCl, 1% Triton X-100, protease inhibitor cocktail (PI; Roche, Rotkreuz, Switerland), and passed through a high-pressure homogenizer (Emulsiflex-C5; Avestin Inc., Mannheim, Germany). The obtained lysates were spun down at 5000 g for 30 min and supernatants were incubated overnight with Ni-NTA agarose beads (Invitrogen, Basel, Switzerland) at 4 °C. Bound proteins were eluted in 1% NP-40 containing 250 mM imidazole (pH 7.8), analysed by Coomassie-stained SDS–PAGE (sodium dodecyl sulfate-polyacrylamide gel electrophoresis), and quantified by bicinchoninic acid (BCA; Pierce, Rockford, Illinois, USA). The normalization was validated by WB. Recombinant APP-C100-Flag and Notch N100-Flag substrates were also expressed in BL21(DE3) cells, but 100 mM glycine (pH 2.7)/1% NP-40 was used for elution from M2-agarose beads. APP-C100-Flag or APP-C100-His substrate consist of the β-CTF (C99) portion of APP (residues 596-695) fused to C-terminal Flag- or His-tag. The Notch cleavage assay used N100-Flag, a Notch-based substrate corresponding to residues Val-1711 to Glu-1809 from murine Notch-1; this protein segment was also fused to a C-terminal Flag-tag. For convenience in the text we have used APP-C99-Flag or APP-C99-His and NotchΔE-Flag. Western blotting and antibodies Samples from γ-secretase activity assays were run on 4–12% Bis-Tris gels and transferred onto PVDF membranes to detect Aβ, Flag-tagged APP- or Notch intracellular domain (AICD-Flag and NICD-Flag) with Aβ-specific 6E10 (1:1,000; Covance, Berkeley, California, USA) and Flag-specific M2 antibodies (1:1,000; Sigma-Aldrich GmbH, Buchs, Switzerland). Anti-mouse/rabbit/rat IgG conjugated to Alexa 680 were purchased from Invitrogen and the Odyssey infrared imaging system (LICOR) was used to detect the fluorescent signal. Whole cell extracts prepared in 50 mM HEPES buffer containing 1% NP-40 were separated by electrophoresis on NuPAGE Novex 4–12% Bis-Tris Gels (Invitrogen, Carlsbad, California, USA) for SDS–PAGE analysis, transferred onto nitrocellulose membranes and probed with antibodies against APP-CTFs (Sigma-Aldrich GmbH, Buchs, Switzerland.). For detection of NICD, membranes were blocked with 5% milk and incubated overnight with primary antibody Val1744 anti-Notch (Cell Signaling, Bioconcept, Allchwil, Switzerland) at 4 °C. Membranes were washed with 1 × TBST (1 × TBS+0.1% Tween 20) for 15 min and incubated with HRP-conjugated secondary antibodies for 1 h at room temperature. Signal was detected with Super Signal West chemiluminescent substrate (Thermo Scientific, catalogue number 34077). γ-Secretase purification γ-Secretase used in this study was composed of PS1, Aph1aL, NCT and Pen-2, and was purified from 10 l of PB suspension cultures by following the protocol described by Alattia et al. [34] γ-Secretase activity assays γ-Secretase assays using the recombinant APP- or Notch-based substrates were performed as previously reported [35] . Briefly, highly purified γ-secretase were solubilized in 0.2% (wt/vol) CHAPSO, 50 mM HEPES (pH 7.0), 150 mM NaCl, 5 mM MgCl 2 and 5 mM CaCl 2 , and incubated at 37 °C for 4 h with 1 μM substrate, 0.1% (wt/vol) PC, 0.025% (wt/vol) PE. The resulting products, APP intracellular domain AICD-Flag, AICD-His, Aβ, and Notch intracellular domain NICD-Flag were detected with above-described antibodies, or analysed by mass spectrometry. Immunoprecipitation-mass spectrometry analysis of Aβ and AICD Aβ and AICD generated in γ-secretase in vitro assays with purified substrates were analysed as previously described [35] . Briefly, Aβ was IP’d overnight using anti-Aβ antibody 4G8 (Covance, Berkeley, California, USA) and protein G coupled to agarose resin (Roche Applied Science, Penzberg, Germany). For AICD or NICD detection, 12 ml 10% Triton X-100 solution was added after the enzymatic reaction and incubated for 20 min at 55 °C prior to overnight immunoprecipitation at 4 °C with M2-anti Flag resin (Invitrogen) or Protein G (Roche, Mannheim, Germany), coupled with anti-C-terminal AICD antibody. Aβ and AICD-Flag were eluted with 1:20:20 ( v : v : v ) 1% (vol/vol) trifluoroacetic acid:acetonitrile:H 2 O, equally mixed with saturated CHCA (α-cyano 4-hydroxy cinnaminic acid) for Aβ, or sinapic acid for AICD, and analysed by MALDI-TOF mass spectrometry in reflectron or linear mode on an ABI 4800 MALDI-TOF/TOF mass spectrometer (Applied Biosystems, Carlsbad, California, USA). Molecular masses were accurately measured and searched against amino-acid sequences of human APP-C99 with addition of a methionine residue at the N terminus and a Flag tag sequence (C100Flag) or a His-tag sequence (C100His) at the C terminus, or a A692G, E693G, D654N, T714I, V715A, I716V, V717F and L723P substitution. MD simulations and molecular docking We used MD simulations to characterize the TM domain of WT and APP with FAD mutations. In a first step, the NMR structure (PDB code 2LP1 (ref. 27 )) was inserted and equilibrated in a 60 × 60 Å 2 POPC patch [36] to relax the structure in a phospholipid bilayer. The system was solvated in 60 × 60 × 100 Å 2 water box, neutralized through the addition of NaCl at a concentration of 150 mM. After 30 ns, the equilibrated structure was used as initial seed to build the other three mutants (V714A, T715I and V717F) and WT-ligand complex. GSM-1 ligand was parameterized using CGenFF and ParamChem 0.9.6 (ref. 37 ). All MD simulations were performed using NAMD 2.8 engine, with the CHARMM27 force field, including CMAP corrections for the protein and CHARMM36 for the POPC membrane [38] , [39] . TIP3P water parameterization was used to describe the water molecules. The periodic electrostatic interactions were computed using the particle-mesh Ewald (PME) summation with a grid spacing <1 Å. All systems were equilibrated for 30 ns at 300 K. Free molecular dynamics were performed up to 100 ns with a 2 fs integration time step using the RATTLE algorithm applied to all bonds. Constant temperature (300 K) was imposed by using Langevin dynamics, with damping coefficient of 1.0 ps. Constant pressure of 1 atm was maintained with a Langevin piston dynamics, 200 fs decay period and 50 fs time constant. GSM-1 was docked on WT and APP mutants using SWISSDock [40] , [41] and BSP-SLIM [42] ; independently both approaches produced similar poses. As these algorithms do not account for the presence of the membrane, we discarded all unphysical docking poses, for example, the GSM-1 hydroxyl being buried in the hydrophobic membrane core. The conformation with the lowest energy was then selected for each system. How to cite this article: Dimitrov, M. et al. Alzheimer’s disease mutations in APP but not γ-secretase modulators affect epsilon-cleavage-dependent AICD production. Nat. Commun. 4:2246 doi: 10.1038/ncomms3246 (2013).